Granular acoustic switches and logic elements Electrical flow control devices are fundamental components in electrical appliances and computers; similarly, optical switches are essential in a number of communication, computation and quantum information-processing applications. An acoustic counterpart would use an acoustic (mechanical) signal to control the mechanical energy flow through a solid material. Although earlier research has demonstrated acoustic diodes or circulators, no acoustic switches with wide operational frequency ranges and controllability have been realized. Here we propose and demonstrate an acoustic switch based on a driven chain of spherical particles with a nonlinear contact force. We experimentally and numerically verify that this switching mechanism stems from a combination of nonlinearity and bandgap effects. We also realize the OR and AND acoustic logic elements by exploiting the nonlinear dynamical effects of the granular chain. We anticipate these results to enable the creation of novel acoustic devices for the control of mechanical energy flow in high-performance ultrasonic devices. The ability to dynamically control the transmission of mechanical energy allows the development of novel materials and devices that can actively control the flow of acoustic or thermal information. Such devices can be used in improved thermoelectric systems, communication lines and medical ultrasonic imaging. In analogy with electrical and optical counterparts [1] , [2] , [3] , a growing number of papers have proposed and tested acoustic diodes [4] , [5] , [6] , [7] , [8] , [9] . For example, directional acoustic propagation was shown using a superlattice coupled with a nonlinear material [4] . Other research exploited nonlinear bifurcation phenomena to realize a tunable acoustic diode [5] . In all these devices, the directional propagation relies on the passive properties of the systems studied; the obvious extension is to create an acoustic counterpart to an electrical or optical flow control device, allowing for active control of energy transfer. Recently, an acoustic circulator was realized, in which the direction of sound transmission can be actively selected [10] , [11] . However, this device requires fluid flow and cannot be controlled by external acoustic waves. Surface acoustic wave logic devices have been realized by using the addition or subtraction of out-of-phase sources [12] . Logic circuits based on a single mechanical resonator have also been demonstrated in high-vacuum and low-temperature environments [13] . Furthermore, a sonic crystal switch based on the destructive interference of two signals was reported [14] . However, the performance of these devices is limited to a relatively narrow band of frequencies of operation. There have been theoretical attempts to design and demonstrate thermal switches and logic gates that manipulate phonons [15] , [16] , but acoustic switches capable of actively controlling a wide frequency range of acoustic signals via an external input remain elusive. An experimental realization of such acoustic switches and logic gates has not been demonstrated, although relevant notions have been theoretically proposed [5] , [17] , [18] . One-dimensional granular chains have been extensively studied for the past two decades, as they present a practically realizable example of a discrete system with a nonlinear contact relation due to the particles’ contact geometry [19] , [20] , [21] , [22] , [23] . The force–displacement law between two solid spheres in contact is governed by a 3/2-power (Hertzian) interaction and has zero tensile force [24] . When two identical spheres are held in contact by static precompression, the stiffness of the Hertzian interaction can be linearized to: which is deformation dependent. Here F is the compression force, δ is the particle’s deformation and δ 0 is the deformation at static equilibrium. is an elastic parameter characterizing the geometric and elastic properties of the medium. The parameters R , E and ν here denote the radius, Young’s modulus and the Poisson ratio of the spheres, respectively. When a high-amplitude acoustic wave of a certain control frequency ( f c ) propagates in the granular chain, it induces large deformations between the particles and the interparticle stiffness varies appreciably according to equation (1). This dynamically varying stiffness mechanism can be used to control acoustic waves when it is combined with the presence of acoustic frequency bandgaps. Similarly to what is seen in traditional phonon theory [25] , [26] , [27] , a chain of compressed spheres presents an acoustic band structure for weak travelling waves, with high frequencies decaying exponentially as they travel through the crystal [21] . The cutoff frequency f cutoff of the chain’s pass band is determined to be for sphere mass M and static precompression force F 0 . If an input wave f o lies above the cutoff frequency f cutoff , it normally would not propagate through the crystal, corresponding to an off state ( Fig. 1a ). However, should f c be turned on as well, the interactions between the two waves will generate harmonics that are linear combinations of the two frequencies ( nf o ± mf c , where n and m are arbitrary integers), as shown in Fig. 1b . If any of the harmonics’ frequencies lie within the pass band (such as f o − f c and f o −2 f c as shown in Fig. 1b ), they will propagate through the chain. These transmitted waves, in turn, will enable the transmission of waves with frequencies in the bandgap that would otherwise not be transmitted. In particular, the interaction between the frequencies f o − f c and f c will regenerate acoustic waves at f o , previously blocked. Therefore, if the acoustic wave f c is within a suitable frequency range and the amplitude is high enough, the acoustic wave f o will now travel to the end of the chain, corresponding to an on state. 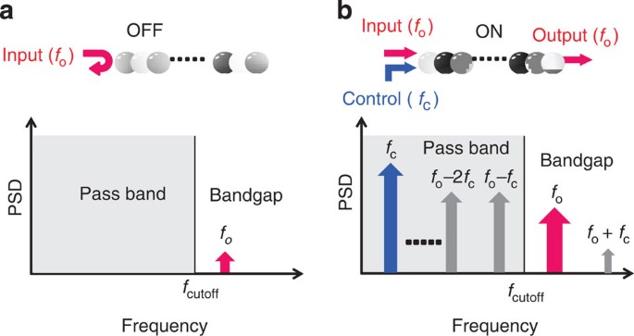Figure 1: Concept of the acoustic granular crystal switch. (a) Off state: the acoustic wavefois above the cutoff frequencyfcutoffand cannot travel. (b) On state: the acoustic wave atfointeracts withfc, generating harmonic waves including one with frequencyfo−fc. Iffo−fcis belowfcutoff, the wave atfocan be reconstructed at the end of the crystal byfcandfo−fc. Figure 1: Concept of the acoustic granular crystal switch. ( a ) Off state: the acoustic wave f o is above the cutoff frequency f cutoff and cannot travel. ( b ) On state: the acoustic wave at f o interacts with f c , generating harmonic waves including one with frequency f o − f c . If f o − f c is below f cutoff , the wave at f o can be reconstructed at the end of the crystal by f c and f o − f c . Full size image On the basis of this principle, here we theoretically analyse, numerically confirm and experimentally implement an acoustic switch based on a nonlinear granular chain, composed of tightly packed solid spheres in Hertzian contact. We show the chain’s ability to act as a switch by modulating an oscillatory acoustic input signal with a second, external signal. We also quantify the transmission efficiency and demonstrate the chain’s ability to act as an AND and an OR logic element. Acoustic switches The experimental frequency response of the chain in terms of the power spectral density (PSD) of transmitted force is shown in Fig. 2a . The peaks in the response curves correspond to the resonances of the chain. The measured cutoff frequency is ~7.4 kHz, which is in agreement with the theoretical prediction. This cutoff is denoted by the vertical dashed line. When we excite the chain with a single harmonic excitation with amplitude a o =0.03 μm and frequency f o =7,660 Hz, we observe that this output frequency does not propagate, as shown by the red curves in Fig. 2b . This corresponds to the off state. 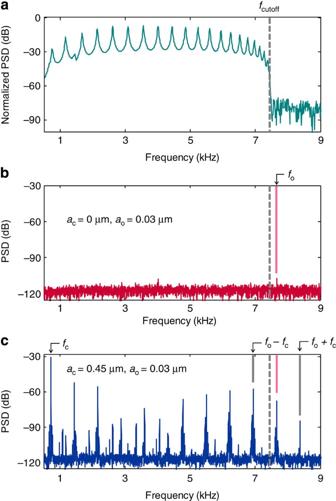Figure 2: Experimental data. (a) The curve shows the normalized transmitted frequency response of the chain. The dashed grey line corresponds to the theoretical cutoff frequency. (b) Off configuration: the acoustic wave atfo(7,660 Hz) cannot propagate. (c) On configuration: when a high-amplitude acoustic wave withac=0.45 μm andfc=720 Hz is added, the transmitted signal is significantly modulated and the wave atfois allowed to propagate. Figure 2: Experimental data. ( a ) The curve shows the normalized transmitted frequency response of the chain. The dashed grey line corresponds to the theoretical cutoff frequency. ( b ) Off configuration: the acoustic wave at f o (7,660 Hz) cannot propagate. ( c ) On configuration: when a high-amplitude acoustic wave with a c =0.45 μm and f c =720 Hz is added, the transmitted signal is significantly modulated and the wave at f o is allowed to propagate. Full size image We then excite the chain with an additional signal at frequency f c =720 Hz and amplitude a c =0.45 μm, on the same order of magnitude as the initial deformation (1.0 μm; Fig. 2c ). When the control signal f c is turned on, the transmitted signal contains harmonics of f c , for example, 2˙ f c and 3˙ f c at 1,440 and 2,160 Hz. In addition, the transmitted signal contains the frequencies of f o − f c (6,940 Hz), f o (7,660 Hz) and f o + f c (8,380 Hz). Compared with the off state in Fig. 2b , the intensity of f o detected at the end of the crystal increases by 40 dB. Thus, by using a strong control acoustic wave, we switch on the acoustic transmission at f o , previously forbidden by the bandgap. The experimental results are in agreement with numerical simulations (see Supplementary Fig. 1 and Supplementary Note 1 ). The PSD of velocity fluctuation of the n th spheres in the chain is normalized by that of the first bead at frequency f o (shown in Fig. 3a ). During the off state, the PSD decays exponentially from the first bead to the last, characteristic of an evanescent wave. However, due to vibration of the mechanical supports in the experimental setup, the acoustic waves are not completely insulated. This effect represents the leakage in our device and is evident from looking at the experimentally determined PSD (red circles in Fig. 3a ), which depart from the simulated values (red line) from the 12th bead onward. In contrast, during the on state, the f o component stops decaying approximately after the fifth bead reaching a steady level, in agreement with the corresponding numerical computations of the system. 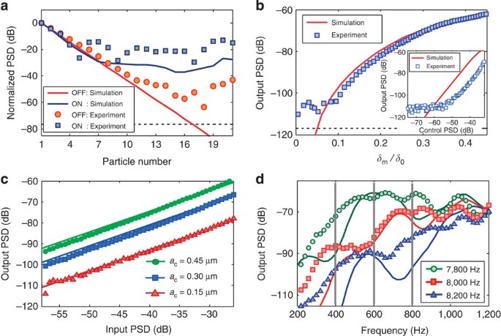Figure 3: PSD of the bead and power transmission. (a) The PSD of the spheres’ velocities normalized by the first bead’s velocity at frequencyfoin the off and on cases. The black dashed line represents the noise floor of the measurement. The continuous curves correspond to the numerical and the dots/squares to the experimental results. (b) PSD of the 7,660 Hz component of the transmitted signal reaching the chains’ boundary. The transmitted amplitude increases with the relative dynamic deformation. The black dashed line denotes the noise floor of the measurement. Inset: relationship between the control and output PSD at frequencyfc=720 Hz. (c) Output PSD as a function of input PSD at frequencyfo=7,660 Hz given three different excitation amplitudesac. (d) Variation of the transmission of the acoustic wave at frequencyfoas a function of the control frequencyfc. Figure 3: PSD of the bead and power transmission. ( a ) The PSD of the spheres’ velocities normalized by the first bead’s velocity at frequency f o in the off and on cases. The black dashed line represents the noise floor of the measurement. The continuous curves correspond to the numerical and the dots/squares to the experimental results. ( b ) PSD of the 7,660 Hz component of the transmitted signal reaching the chains’ boundary. The transmitted amplitude increases with the relative dynamic deformation. The black dashed line denotes the noise floor of the measurement. Inset: relationship between the control and output PSD at frequency f c =720 Hz. ( c ) Output PSD as a function of input PSD at frequency f o =7,660 Hz given three different excitation amplitudes a c . ( d ) Variation of the transmission of the acoustic wave at frequency f o as a function of the control frequency f c . Full size image We quantify the transmission efficiency in terms of the PSD of the f o component at the end boundary. We define the transmitted signal as the maximum dynamic deformation at the boundary (that is, between the last bead and the force sensor) relative to the static deformation ( δ m /δ 0 ) ( Fig. 3b ). Experiments show an on/off ratio larger than 40 dB when the relative dynamic deformation is larger than 0.3. If δ m /δ 0 is less than 0.1, the amplitude of the transmitted f o component due to the switching effect becomes smaller than the acoustic leakage, and this switching effect is no longer attainable. In other words, the switching effect increases with the relative dynamic deformation, thus establishing the nonlinear character of the switch. The relationship between the output PSD at frequency f o and the control PSD at frequency f c is plotted in the inset of Fig. 3b . The output PSD increases gradually with the control PSD, and the experimental results follow this trend of numerical simulations when the control PSD is larger than −60 dB. The slope of the output versus the control PSD is larger than 1 (close to 2, implying that output power is proportional to the square of the control power). This proves the sensitive controllability of acoustic waves with variations of the control signals in our device. To demonstrate the controllability of the system, we plot the relationship between the input and the output PSD at frequency f o given three different excitation amplitudes a c ( Fig. 3c ). The solid lines correspond to the numerical input–output relationship, and we find that the slopes of these parallel lines are 1, which means that the output is in linear relationship with the input. The experimental results are also plotted in the same figure and agree well with the simulation results. It is important to note that the lines can be shifted upwards by introducing a stronger control wave, which implies that the input–output relationship can be actively tuned. This is phenomenologically similar to an electrical transistor, in which the base-collector voltage can control the relationship between the collector current and collector–emitter voltage. When a c increases from 0.30 to 0.45 μm, the line upshift is not as large as the one observed when a c increases from 0.15 to 0.30 μm. Even in the case of a large control amplitude a c , the device still suffers a considerable loss (~40 dB) in signal strength. The loss cannot be decreased much by further increasing the drive amplitude a c because gaps may appear (that is, δ n , n +1 + u n − u n +1 <0) between beads due to strong excitations. When gaps form, the harmonic acoustic waves become distorted and the linear band structure compromised, resulting in a breakdown of our device. From the basic working principles of the acoustic switch presented in Fig. 1 , there should exist a threshold frequency ( f T =f o − f cutoff ) for a given f o . When f c is above f T , the switching effect is expected to occur. To show this threshold, we investigate the dependence of the transmission at f o , by looking at three different frequencies of f o (7,800, 8,000 and 8,200 Hz) at the same amplitude of a o (0.06 μm). Because f c is within the pass band, the transmission at frequency f o varies significantly with f c due to the resonant modes of the 21 beads. We normalize this effect by employing different excitation amplitude a c corresponding to different frequency f c while keeping the dynamic deformation between the last bead and the boundary a constant value ( δ m =0.31 μm). The numerical results (solid curves) and the experimental results (discrete points) of the switch’s transmission with respect to f c are shown in Fig. 3d . The grey vertical lines (400, 600 and 800 Hz) denote the threshold frequencies f T for the three output frequencies f o studied. The qualitative trends of the experiments are captured by the numerical simulations. In Fig. 3d , the transmission response shifts to higher frequencies when f o increases from 7,800 to 8,200 Hz in accordance with our predictions. Instead of a vertical ‘cliff’ response at f T (grey lines in Fig. 3d ), the transmission curves have relatively wide slopes around f T and fluctuate significantly above f T because of the resonances of the chain. In addition, due to the contribution of higher harmonics, there could be considerable transmission even if f c is below f T (for example, the interaction of f o − 2˙f c and 2˙f c can generate the acoustic wave f o as shown in Fig. 1b ). This can be improved by increasing the number of particles in the chain or suppressing the effect of additional harmonics by reducing the dynamic force applied to the chain (see Supplementary Fig. 2 and Supplementary Note 2 for the numerical simulations). The character of f T for the switch is qualitatively analogous to an electrical transistor, in which there exists a threshold voltage V th : when the gate source voltage V g is higher than V th , the conducting channel begins to connect the source and drain of the transistor, allowing a large current to flow. However, unlike an electrical transistor, which remains open when V g is much higher than V th , if the controlling frequency f c increases further up to f cutoff , both the controlling and output acoustic waves at f c and f o are cut off and the switching effect disappears, at which point the switching function is unavailable. Thus, theoretically, the acoustic granular switch is only functional if f c is located within the frequency range f T to f cutoff (that is, in terms of f o , it should be located within the frequency range f cutoff to f c + f cutoff ) and this upper frequency limit of the controlling wave f c acts as a ‘breakdown’ frequency. It is important to note that, while this type of mechanical wave control mechanism is reminiscent of the functionality of an acoustic transistor, the transmitted output wave in our setup is much weaker than the control wave, not the other way around [18] . This implies that the granular switch presented in this study is not capable of amplifying signals like an electric transistor. Acoustic logic elements On the basis of our acoustic switch, we next demonstrate the realization of OR ( ∪ ) and AND (∩) logic elements by using dual-control signals. We use three function generators and produce sinusoidal excitations with three frequencies at the same time. Two strong controlling excitations at f c1 =720 Hz and f c2 =880 Hz and one weak excitation at f o =7,660 Hz are chosen. For the piezo actuator, the amplitudes of the components at these three frequencies are a c1 = a c2 =0.40 μm and a o =0.03 μm, respectively. The experimental results of the logic elements AND and OR are reported in Fig. 4 . The strong excitation states (on and off) correspond to logic inputs (Boolean states 1 and 0). Because of nonlinear interactions between 720 and 880 Hz, the two frequencies will combine to produce an extra signal at 1,600 Hz (720+880 Hz), which creates the logical AND output. Because the acoustic wave at 7,660 Hz is located out of the pass band, when A=0 and B=0 , the acoustic wave at 7,660 Hz cannot propagate. However, if either input of 720 or 880 Hz is provided, the 7,660 Hz signal is switched on, creating a logical OR . Beyond fundamental two-bit logic calculation, it is possible to realize multi-bit logic operation on a single structure by using multiple control frequencies or introducing phase information [13] , [28] . For example, by adding anti-phase signals at f c1 and f c2 , the NOT operation can be enabled due to destructive interference, and thus, NOR and NAND functions can also be realized. If we introduce a third control frequency at f c3 below f T , the operations of A∩B∩C and (A ∪ B)∩C can be realized at frequencies f c1 + f c2 + f c3 and f o + f c3 , respectively. Nevertheless, as a limitation of the present approach, we recognize that it does not feature the trait of cascadability associated with classical logic devices [3] . 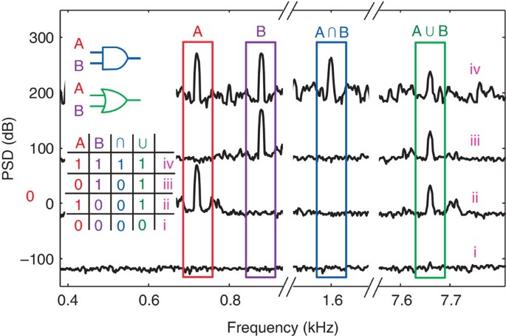Figure 4: Acoustic logic elements. The acoustic logic elements OR and AND are realized by employing two different controlling frequencies. The PSD curves are shifted vertically by 100 dB to ease visualization. Figure 4: Acoustic logic elements. The acoustic logic elements OR and AND are realized by employing two different controlling frequencies. The PSD curves are shifted vertically by 100 dB to ease visualization. Full size image We have shown that, in a continuously driven granular chain, a non-propagating evanescent wave can be transformed into a propagating one by combining the presence of a bandgap with nonlinear wave mixing in the presence of a control frequency. We thus realize an acoustic transistor switch, which enables the control of one acoustic wave by another. On the basis of this, the acoustic logic elements OR and AND were demonstrated by use of dual-frequency signals and monitoring different output frequencies. These findings make it now possible to design advanced acoustic devices, which can dynamically control acoustic waves in a tunable and efficient manner. Although the concept of the acoustic switch has been realized in granular media in this study, the same principle can be applicable in other materials or systems interweaving the principal features of nonlinearity and spatial periodicity. Using nonlinear effects, we can further explore other gating options aside from the ones considered here. The tunability and robustness of the phenomena proposed here suggest their potential extension to higher dimensions, particularly towards the blocking, routing and other related operations of acoustic waves, similarly to what has been theoretically proposed, for example, in nonlinear optics [29] . Experimental setup The particle chain studied is composed of 21 chrome steel beads linearly aligned (see Supplementary Fig. 3 for details). The mass M , radius R , the nominal values of Young’s modulus E and the Poisson’s ratio ν of the spheres are 28.2 g, 9.525 mm, 200 GPa and 0.3, respectively. The reported values of E and ν are standard specifications [30] . The spherical particles are horizontally aligned and supported by four polytetrafluoroethylene (PTFE) rods to reduce friction. The positions of these PTFE rods are precisely controlled by linear stages to restrict the lateral motions of beads with the minimal clearance between the beads and the rods. The chain is precompressed with a force ( F 0 ) of 10 N, which gives an initial deformation δ 0 of 1.0 μm. Two sinusoidal signals from function generators (at frequencies f c and f o ) are added together, amplified and used to drive a piezoelectric actuator at one end of the chain. The actuator excites the chain in the axial direction from one end. To gain further insight as to the propagation of wave energy through the chain, we measure the dynamic force at the boundary by force sensor (PCB 208C01). We use a Laser Doppler Vibrometer (Polytec OFV 534), which measures the axial velocity fluctuation of each particle and is scanned across the chain by a moving stage [31] . The signal is further analysed by a spectrum analyser to obtain the PSD of velocity fluctuations. The PSD of the n th particle at f o is normalized by subtracting that value of the first particle. The displacements of the beads are obtained by numerical integration of the measured velocities. The input force is indirectly measured from the measured displacements of the actuator u 0 and first bead u 1 . Both the output force and velocity signals acquired are then analysed by a network analyzer (Agilent 4395a) and a spectrum analyzer (Stanford Research SR785). Numerical approach The particles have a uniform mass M and interparticle Hertzian coefficients A n,n +1 between the n th and ( n +1)th particles. The full equation of motion for the spherical chain with dissipation and excitation of the sum of two sinusoidal waves can be written as [5] : where u n is the displacement of the n th bead ( u 0 and u 22 denote the actuator’s and sensor’s displacements); δ n , n +1 =( F 0 / A n , n +1 ) 2/3 is the deformation at static equilibrium between the n th and ( n +1)th particles; and a c ( a o ) and f c ( f o ) are the amplitude and frequency of the control (output) sinusoidal excitations of the actuator. The Hertzian coefficient is given by , where R n is the radius of the n th bead ( R 0 and R 22 are approximated to ∞). The bracket, defined by [ x ] + =max (0 , x ), denotes that there are no tensile forces between the particles. The dissipation factor τ (5 ms) was determined by measuring wave propagation decay in experiments and determining a parameter that matched the results numerically [5] . These equations of motion were numerically integrated using Matlab’s ODE113 routine. How to cite this article: Li, F. et al. Granular acoustic switches and logic elements. Nat. Commun. 5:5311 doi: 10.1038/ncomms6311 (2014).